The role and assembly mechanism of nucleoprotein in influenza A virus ribonucleoprotein complexes The nucleoprotein of negative-strand RNA viruses forms a major component of the ribonucleoprotein complex that is responsible for viral transcription and replication. However, the precise role of nucleoprotein in viral RNA transcription and replication is not clear. Here we show that nucleoprotein of influenza A virus is entirely dispensable for replication and transcription of short viral RNA-like templates in vivo , suggesting that nucleoprotein represents an elongation factor for the viral RNA polymerase. We also find that the recruitment of nucleoprotein to nascent ribonucleoprotein complexes during replication of full-length viral genes is mediated through nucleoprotein–nucleoprotein homo-oligomerization in a ‘tail loop-first’ orientation and is independent of RNA binding. This work demonstrates that nucleoprotein does not regulate the initiation and termination of transcription and replication by the viral polymerase in vivo , and provides new mechanistic insights into the assembly and regulation of viral ribonucleoprotein complexes. The genomes of all negative-strand RNA viruses (NSVs) are coated by the viral nucleoprotein (NP). Together with the viral RNA-dependent RNA polymerase, these ribonucleoprotein (RNP) complexes form the minimal functional unit for all viral transcription and replication. Although a great deal is known about the functionality of the viral polymerase, the role of NP remains unclear. In addition, little is known about the mechanism of NP assembly into RNPs, or how the polymerase is able to read through NP-bound RNA templates. The atomic structures of NP from different NSVs [1] have revealed two prominent common features, namely a positively charged RNA-binding cleft and the presence of extensive contacts between neighbouring NP molecules, suggesting at least some commonality in function and mechanism. The genome of influenza A virus comprises eight single-stranded negative sense RNA (vRNA) segments [2] . Each genome segment is associated with one heterotrimeric viral RNA-dependent RNA polymerase and multiple copies of NP, forming a viral genomic (v)RNP complex that serves as the template for both transcription and replication [3] . Transcription is initiated with a 10- to 13-nucleotide-long capped primer that is endonucleolytically cleaved from host cellular mRNA [4] , [5] , [6] , and is prematurely terminated by polyadenylation at an oligo(U) sequence near the 5′-end of each vRNA through a stuttering mechanism [7] , [8] , [9] . In contrast, replication initiates de novo and generates a full-length copy of the template RNA [10] . The distinct structures of the positive sense RNAs suggest that the initiation and termination mechanisms for vRNA-templated replication and transcription may be coupled, that is, initiation by cap-snatching is coupled to polyadenylation and de novo initiation is coupled to suppression of premature termination. The role of NP during transcription and replication of the influenza virus genome has long remained an enigma. NP binds RNA with high affinity in a sequence-independent manner [11] , [12] , most likely through the positively charged cleft identified in the atomic structure between the head and body domains [13] , [14] . In addition, the structure revealed the presence of a tail loop by which NP molecules self-associate into oligomeric structures, which has been shown by mutagenesis to be required for RNP activity [15] . NP has also been shown biochemically to interact with polymerase subunits PB1 and PB2 [16] , but information on the interaction domains is limited [17] . It is generally thought that during replication the 5′ terminus of the nascent transcript is bound sequence-specifically and cotranscriptionally by ‘free’ polymerase, which then serves as a nucleation step for the sequence-independent sequential encapsidation of the transcript by NP [3] , [13] , [18] , [19] . Although the viral polymerase cannot replicate full-length genomic RNA in the absence of NP, it has previously been shown in vitro and, more recently, in vivo that replication of short RNA templates can occur in the absence of NP [20] , [21] , [22] , [23] , [24] . Binding of NP in vitro was shown to melt the secondary structure of an artificial mini vRNA of 81 nucleotides and it was suggested that one role of NP may be to facilitate RNA transcription [11] . Indeed, it has previously been proposed that NPs may have a central role in genome replication by supporting the elongation of nascent transcripts [20] , [25] . Besides this structural role in organizing the RNP complex, NP has been implicated in the regulation of transcription and replication of influenza virus, as several temperature-sensitive NP mutations have been identified that result in defective replication at non-permissive temperatures [26] , [27] . Although several models have been proposed (reviewed in Portela and Digard [19] ), the mechanism behind this role is unclear. More recently, the stabilization model proposed that the synthesis of cRNA or mRNA from the virion-derived vRNPs is stochastic, but that the expression of both polymerase and NP are required for the stabilization (and replication) of cRNA [28] . In support of this model, our laboratory has recently shown that the RNA-binding activity of NP is crucial for its role in stabilizing cRNA, whereas both RNA binding and NP oligomerization are needed to support replication [29] . Evidence which shows that the interaction of viral proteins with cellular factors is required for efficient viral transcription and replication has been accumulating [30] , [31] . NP has been shown to interact with numerous cellular factors; most notably, it has been suggested that NP is maintained as a monomer by binding to importin α5 while retaining its RNA-binding activity, whereas UAP56 has been proposed to act as a chaperone to facilitate the binding of NP to RNA [30] , [32] , [33] . The minichromosome maintenance replicative helicase complex has been shown to be required for cRNA synthesis in vivo and to stimulate the elongation of nascent cRNA in vitro [25] , [34] . Minireplicon systems, in which artificial, genome-like reporter RNAs are used as model templates that can be replicated and transcribed in vivo by coexpressed viral polymerase and NP, have been available for over two decades. The authenticity of this approach is demonstrated by the rescue of recombinant influenza virus through the simultaneous generation of eight recombinant RNPs in vivo [35] , [36] . Here we have used the minireplicon system with short influenza A virus vRNA-like templates to show that NP has no role in the regulation of in vivo RNP initiation or termination activity. Our data support the view that the template-associated NP is an essential cofactor required for full processivity of the viral RNA-dependent RNA polymerase during replication of the viral genome. We further find that the cotranscriptional addition of NP to nascent vRNA is mediated unidirectionally by NP homo-oligomerization independently of RNA binding. Micro vRNP-like complexes lacking NP are active in vivo Recently, Resa-Infante et al. [21] described the in vivo replication of a micro 46-nucleotide-long influenza vRNA-like RNA in the absence of NP. To investigate what role, if any, NP has in the regulation of transcription and replication, we constructed a series of short genome segments based on gene segment 5 by internal deletions, minimally retaining the conserved 3′ and 5′ termini and the oligo(U) stretch near to the 5′ terminus ( Supplementary Fig. S1 ). Following in vivo RNP reconstitution, the accumulation of the negative and positive sense viral RNA was analysed by primer extension ( Supplementary Table S1 ). We found that a microgenome segment of 47 nucleotides in length can be replicated efficiently by the viral RNA polymerase in the absence of NP ( Fig. 1a ), in agreement with Resa-Infante et al. [21] In addition, RNA with a 5′-terminal extension, corresponding to mRNA, was also detected both in the presence and absence of NP. Using longer RNA templates we determined that the viral polymerase is also able to efficiently replicate and transcribe a 76-nucleotide-long template in the absence of NP. However, NP was found to be essential for the replication of templates of 101 nucleotides and longer ( Fig. 1a ). To further characterize the RNA species accumulating during replication and transcription of microgenome segments in the presence and absence of NP, total RNA samples were separated by oligo(dT) chromatography and the fractions were then analysed by primer extension ( Fig. 1b ). No differences were observed in the character of the RNA species accumulating in the presence or absence of NP. RNA that was bound to oligo(dT) and is thus polyadenylated, was found to possess a 5′-terminal extension, as expected of viral mRNA. In contrast, vRNA, which is not polyadenylated, did not bind to oligo(dT). To determine whether NP has any role in replication and transcription of micro RNA templates, titrations of NP and polymerase were carried out. These data revealed that the presence of increasing concentrations of NP stimulates replication and transcription of a 76-nucleotide-long template ( Supplementary Fig. S2 ), especially at lower polymerase concentrations. Although we do not currently know the mechanism for this stimulation, significant levels of replication and transcription were detected in the absence of NP at all concentrations of polymerase tested. Overall, therefore, these data suggest that NP is not essential for the activity of reconstituted micro RNPs containing templates of up to 76 nucleotides in length, neither in the initiation nor termination of replication or transcription, or any possible coupling between these activities. However, NP is required for the transcription and replication of longer templates, suggesting that NP primarily has a role as an elongation factor. 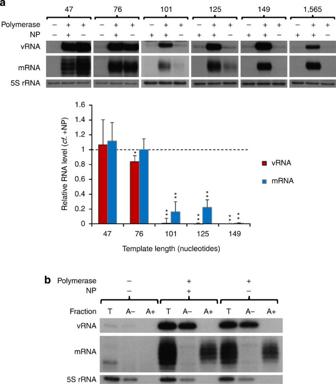Figure 1: The role of NP in the activity of vRNP-like complexes. (a) The accumulation of vRNA and mRNA followingin vivoreconstitution of vRNPs from trimeric polymerase, and varying lengths of segment 5-based vRNA-like templates in the presence or absence of wild-type (wt) NP were analysed by primer extension. PA was omitted as a negative control. The lengths of the vRNA-like gene segments (in nucleotides) are indicated above. The 1,565-nucleotide-long template represents full-length segment 5 containing mutations to prevent expression of NP. Quantification was performed by phosphorimage analysis of at least three independent experiments. Analysis of the 5S rRNA levels served as an internal control. RNA levels detected in the negative control were set to 0. A graph depicting the vRNA and mRNA levels accumulating from each construct in the absence of NP relative to those accumulating in the presence of NP is shown. Error bars indicate s.e.m., and the asterisks indicate a significant difference from 1 (one samplettest; *P<0.05, **P<0.01). (b) Primer extension analysis of RNA samples separated by oligo(dT) chromatography fromin vivoreconstituted RNPs with the 76-nucleotide-long template in the presence or absence of wt NP. Fractions: T, total RNA; A−, RNA not bound to oligo(dT); A+, RNA bound to oligo(dT). Figure 1: The role of NP in the activity of vRNP-like complexes. ( a ) The accumulation of vRNA and mRNA following in vivo reconstitution of vRNPs from trimeric polymerase, and varying lengths of segment 5-based vRNA-like templates in the presence or absence of wild-type (wt) NP were analysed by primer extension. PA was omitted as a negative control. The lengths of the vRNA-like gene segments (in nucleotides) are indicated above. The 1,565-nucleotide-long template represents full-length segment 5 containing mutations to prevent expression of NP. Quantification was performed by phosphorimage analysis of at least three independent experiments. Analysis of the 5S rRNA levels served as an internal control. RNA levels detected in the negative control were set to 0. A graph depicting the vRNA and mRNA levels accumulating from each construct in the absence of NP relative to those accumulating in the presence of NP is shown. Error bars indicate s.e.m., and the asterisks indicate a significant difference from 1 (one sample t test; * P <0.05, ** P <0.01). ( b ) Primer extension analysis of RNA samples separated by oligo(dT) chromatography from in vivo reconstituted RNPs with the 76-nucleotide-long template in the presence or absence of wt NP. Fractions: T, total RNA; A−, RNA not bound to oligo(dT); A+, RNA bound to oligo(dT). Full size image Monomeric NP supports activity of mini vRNP-like complexes NP has been found to self-assemble into oligomers through a tail loop structure (residues 402–428) mediating the interaction of neighbouring molecules [13] , [14] , [15] . The identities of the essential molecular contacts between neighbouring NPs, notably R416 and E339, and the relevance of the interaction for vRNP function, have been confirmed through mutagenesis studies [13] , [15] , [37] . As each NP in the RNP structure is believed to be associated with approximately 24 nucleotides [38] , [39] , we speculated that the addition of monomeric NP may suffice for the replication and transcription of a 101-nucleotide-long template. Indeed, the addition of oligomerization mutant NP R416A ( Fig. 2a ) or E339A ( Fig. 2b ) promoted replication and transcription of the 101-nucleotide-long template, as well as or better than wild-type NP. To our surprise, templates up to 221 nucleotides long were also replicated as well in the presence of the oligomerization mutant NP as in the presence of wild-type NP. Intriguingly, despite wild-type levels of replication, mRNA transcribed from the 149- to 221-nucleotide-long templates in the presence of mutant NP accumulated to only ~50% compared with the level achieved in the presence of wild-type NP. Replication and transcription of a 246-nucleotide-long template were significantly reduced in the presence of mutant NP compared with replication and transcription in the presence of wild-type NP, and they were negligible for templates of 287 nucleotides and longer. Similar results were obtained with double-mutant NP E339A/R416A ( Fig. 2c ). It should be pointed out that although the expression level ( Supplementary Fig. S3 ) and subcellular localization ( Supplementary Fig. S4 ) of the oligomerization mutant NPs were shown to be similar to wild-type NPs, we found that at lower concentrations oligomerization mutant NP R416A was less efficient than wild-type NPs at supporting replication and transcription ( Supplementary Fig. S5 ). Overall, we find that non-oligomerizing mutant NP supports the replication and transcription of intermediate-length templates. 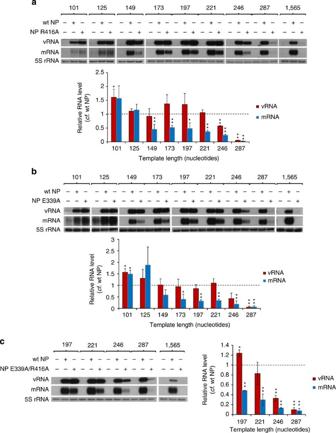Figure 2: The role of NP oligomerization in the activity of vRNP-like complexes. The accumulation of vRNA and mRNA followingin vivoreconstitution of vRNPs from trimeric polymerase and varying lengths of segment 5-based vRNA-like templates in the presence of wild type (wt) or oligomerization mutant (R416A (a), E339A (b) or E339A/R416A (c)) NP were analysed by primer extension. NP was omitted as a negative control. The lengths of the vRNA-like gene segments (in nucleotides) are indicated above. The 1,565-nucleotide-long template represents full-length segment 5 containing mutations to prevent expression of NP. Quantification was performed by phosphorimage analysis of at least three independent experiments. Analysis of the 5S rRNA levels served as an internal control. RNA levels detected in the negative control were set to 0. Graphs depicting the vRNA and mRNA levels accumulating from each construct in the presence of mutant NP relative to those accumulating in the presence of wt NP are shown. Error bars indicate s.e.m., and the asterisks indicate a significant difference from 1 (one samplettest; *P<0.05, **P<0.01). Figure 2: The role of NP oligomerization in the activity of vRNP-like complexes. The accumulation of vRNA and mRNA following in vivo reconstitution of vRNPs from trimeric polymerase and varying lengths of segment 5-based vRNA-like templates in the presence of wild type (wt) or oligomerization mutant (R416A ( a ), E339A ( b ) or E339A/R416A ( c )) NP were analysed by primer extension. NP was omitted as a negative control. The lengths of the vRNA-like gene segments (in nucleotides) are indicated above. The 1,565-nucleotide-long template represents full-length segment 5 containing mutations to prevent expression of NP. Quantification was performed by phosphorimage analysis of at least three independent experiments. Analysis of the 5S rRNA levels served as an internal control. RNA levels detected in the negative control were set to 0. Graphs depicting the vRNA and mRNA levels accumulating from each construct in the presence of mutant NP relative to those accumulating in the presence of wt NP are shown. Error bars indicate s.e.m., and the asterisks indicate a significant difference from 1 (one sample t test; * P <0.05, ** P <0.01). Full size image RNA binding by NP is crucial for vRNP complex activity NP, in the context of the RNP, is known to bind the resident polymerase and template RNA [12] , [16] , [37] . To study whether the RNA-binding activity of NP is required for its role in supporting the RNP activity, we examined whether NP lacking RNA-binding activity could promote replication of intermediate-length templates. For this purpose, we used NP with mutations at four of the positively charged amino acids in the proposed RNA-binding groove, NP G1(4). The RNA-binding affinity of NP G1(4) has previously been shown to be too low to be determined by surface plasmon resonance, yielding only a weak response even at a high concentration (6.25 μM) of NP G1(4), in contrast to the high RNA-binding affinity of wild-type NP, which was shown to have a dissociation constant ( K D ) of 16.5 nM [29] . In addition, NP G1(4) was shown to possess only residual activity in supporting full-length viral gene replication [29] . As shown in Fig. 3 , we found that NP G1(4) supported replication of the 101- to 149-nucleotide-long templates very weakly (10–30% compared with wild-type NPs). Only barely detectable replication or transcription of templates longer than 149 nucleotides was observed in the presence of the RNA-binding mutant NP G1(4). Interestingly, we observed that the RNA-binding mutant NP G1(4) was able to support transcription of the 101-nucleotide template. In general, we conclude that the RNA-binding activity of NP is important for its role in supporting replication, in agreement with previous observations [27] . 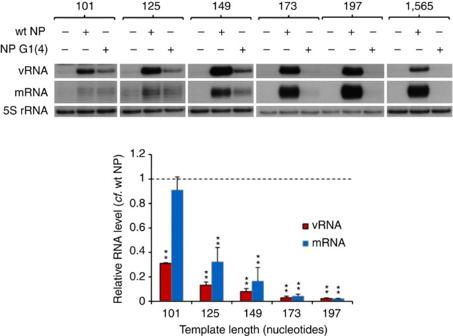Figure 3: The role of RNA-binding by NP in the activity of vRNP-like complexes. The accumulation of vRNA and mRNA followingin vivoreconstitution of vRNPs from trimeric polymerase and varying lengths of segment 5-based vRNA-like templates in the presence of wild type (wt) or RNA-binding mutant (G1(4)) NP was analysed by primer extension. NP was omitted as a negative control. The lengths of the vRNA-like gene segments (in nucleotides) are indicated above. The 1,565-nucleotide-long template represents full-length segment 5 containing mutations to prevent expression of NP. Quantification was performed by phosphorimage analysis of three independent experiments. Analysis of the 5S rRNA levels served as an internal control. RNA levels detected in the negative control were set to 0. A graph depicting the vRNA and mRNA levels accumulating from each construct in the presence of mutant NP relative to those accumulating in the presence of wt NP is shown. Error bars indicate s.e.m., and the asterisks indicate a significant difference from 1 (one samplettest; **P<0.01). Figure 3: The role of RNA-binding by NP in the activity of vRNP-like complexes. The accumulation of vRNA and mRNA following in vivo reconstitution of vRNPs from trimeric polymerase and varying lengths of segment 5-based vRNA-like templates in the presence of wild type (wt) or RNA-binding mutant (G1(4)) NP was analysed by primer extension. NP was omitted as a negative control. The lengths of the vRNA-like gene segments (in nucleotides) are indicated above. The 1,565-nucleotide-long template represents full-length segment 5 containing mutations to prevent expression of NP. Quantification was performed by phosphorimage analysis of three independent experiments. Analysis of the 5S rRNA levels served as an internal control. RNA levels detected in the negative control were set to 0. A graph depicting the vRNA and mRNA levels accumulating from each construct in the presence of mutant NP relative to those accumulating in the presence of wt NP is shown. Error bars indicate s.e.m., and the asterisks indicate a significant difference from 1 (one sample t test; ** P <0.01). Full size image The role of NP is conserved for different vRNP templates To confirm that the data presented above are not peculiar to the particular set of templates used, which are based on gene segment 5, representative minigenome constructs based on gene segment 8 were also analysed. In vivo replication and transcription of segment 8-based vRNA templates 60, 172 or 890 nucleotides in length ( Supplementary Fig. S1 ), the latter representing the full-length genome segment, were compared in the presence or absence of wild-type and mutant NP ( Fig. 4 ). We found that the accumulation levels of vRNA and mRNA from these templates were not necessarily the same as those from the segment 5-based gene segments. For instance, replication and transcription of the segment 8-based 172-nucleotide-long template in the presence of NP R416A was significantly reduced compared with that of the segment 5-based 173-nucleotide-long template. We propose that this may be due to the different templates having different secondary structures. However, overall, these data confirmed that (1) micro vRNA templates can be replicated and transcribed efficiently in the absence of NP, whereas replication and transcription of even the shortest full-length genome segment requires wild-type NP; (2) oligomerization of NP is non-essential for replication of intermediate-length vRNA templates, but their transcription is partially inhibited by mutations in oligomerization domains of NP; and (3) the RNA-binding activity of NP is critical to the role of NP in RNP activity. 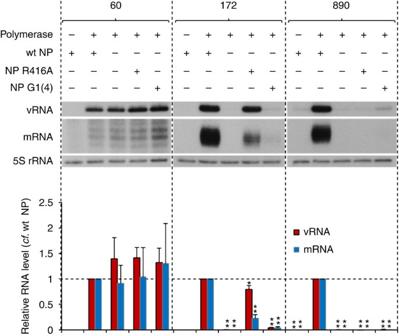Figure 4: The conservation of the role of NP in the activity of vRNP-like complexes. The accumulation of vRNA and mRNA followingin vivoreconstitution of vRNPs from trimeric polymerase and varying lengths of segment 8-based vRNA-like templates in the presence or absence of wild type (wt) or mutant (oligomerization mutant R416A or RNA-binding mutant G1(4)) NP were analysed by primer extension. PA was omitted as a negative control. The lengths of the vRNA-like gene segments (in nucleotides) are indicated above. The 890-nucleotide-long template represents full-length segment 8. Quantification was performed by phosphorimage analysis of three independent experiments. Analysis of the 5S rRNA levels served as an internal control. RNA levels detected in the negative control were set to 0. A graph depicting the vRNA and mRNA levels accumulating from each construct in the absence of NP or in the presence of mutant NP relative to those accumulating in the presence of wt NP is shown. Error bars indicate s.e.m., and the asterisks indicate a significant difference from 1 (one samplettest; *P<0.05, **P<0.01). Figure 4: The conservation of the role of NP in the activity of vRNP-like complexes. The accumulation of vRNA and mRNA following in vivo reconstitution of vRNPs from trimeric polymerase and varying lengths of segment 8-based vRNA-like templates in the presence or absence of wild type (wt) or mutant (oligomerization mutant R416A or RNA-binding mutant G1(4)) NP were analysed by primer extension. PA was omitted as a negative control. The lengths of the vRNA-like gene segments (in nucleotides) are indicated above. The 890-nucleotide-long template represents full-length segment 8. Quantification was performed by phosphorimage analysis of three independent experiments. Analysis of the 5S rRNA levels served as an internal control. RNA levels detected in the negative control were set to 0. A graph depicting the vRNA and mRNA levels accumulating from each construct in the absence of NP or in the presence of mutant NP relative to those accumulating in the presence of wt NP is shown. Error bars indicate s.e.m., and the asterisks indicate a significant difference from 1 (one sample t test; * P <0.05, ** P <0.01). Full size image Monomeric NP is incorporated into mini vRNP complexes To address the question whether non-oligomerizing mutant NP is incorporated into progeny RNP during replication of intermediate-length templates, we carried out RNP reconstitution experiments with the 221-nucleotide template in the presence of his-tagged PA, and we analysed the constituents of complexes copurified during nickel affinity chromatography ( Fig. 5a ). Western blot and primer extension analyses clearly demonstrated the copurification of wild-type or non-oligomerizing NP and vRNA, providing evidence for the assembly of RNP complexes. We also examined the requirement for active trimeric polymerase by RNP reconstitution experiments carried out in the presence or absence of PA ( Fig. 5b ), or in the presence of wild-type PB1 or PB1 with a double mutation in the conserved SDD motif of the active site ( Fig. 5c ). As expected, wild-type and non-oligomerizing mutant NPs were only able to support replication and transcription in the presence of active trimeric polymerase. Therefore, we conclude that replication and transcription of intermediate-length templates is dependent on the assembly of active polymerase and wild-type or non-oligomerizing mutant NPs into RNPs. 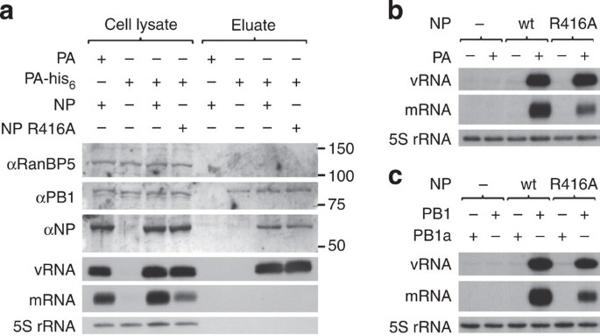Figure 5: Components assembled in active vRNP-like complexes. (a) The proteins and RNA coisolated during nickel affinity chromatography of vRNPs reconstitutedin vivofrom trimeric polymerase (his-tag on PA) and the 221-nucleotide-long vRNA-like template in the presence of wild type (wt) or oligomerization mutant (R416A) NP were analysed by western blot and primer extension, respectively. The use of untagged PA or the omission of NP served as negative controls. The expression of comparable levels of NP, PB1, vRNA and mRNA was confirmed in the cell lysates; RanBP5 and 5S rRNA were detected as loading controls. vRNP components coisolated with PA-his6were detected in the eluates of nickel affinity chromatography. (b,c) Primer extension analysis of the accumulation of vRNA and mRNA derived fromin vivoreconstituted vRNPs with the 221-nucleotide-long template in the presence or absence of PA (b) or in the presence of wt or inactive mutant (D445A/D446A) PB1 (c) and wt or oligomerization mutant (R416A) NP. NP was omitted as a negative control. Analysis of the 5S rRNA levels served as an internal control. Figure 5: Components assembled in active vRNP-like complexes. ( a ) The proteins and RNA coisolated during nickel affinity chromatography of vRNPs reconstituted in vivo from trimeric polymerase (his-tag on PA) and the 221-nucleotide-long vRNA-like template in the presence of wild type (wt) or oligomerization mutant (R416A) NP were analysed by western blot and primer extension, respectively. The use of untagged PA or the omission of NP served as negative controls. The expression of comparable levels of NP, PB1, vRNA and mRNA was confirmed in the cell lysates; RanBP5 and 5S rRNA were detected as loading controls. vRNP components coisolated with PA-his 6 were detected in the eluates of nickel affinity chromatography. ( b , c ) Primer extension analysis of the accumulation of vRNA and mRNA derived from in vivo reconstituted vRNPs with the 221-nucleotide-long template in the presence or absence of PA ( b ) or in the presence of wt or inactive mutant (D445A/D446A) PB1 ( c ) and wt or oligomerization mutant (R416A) NP. NP was omitted as a negative control. Analysis of the 5S rRNA levels served as an internal control. Full size image NP recruitment to RNP complexes is oligomerization-mediated It has been proposed that specific binding of the viral polymerase to the 5′-terminal sequences of nascent vRNAs may act as a nucleation signal for the assembly of progeny RNP by sequential association of NP, possibly mediated through oligomerization [3] , [13] , [18] , [19] . We hypothesized that if this was the case, NP assembly on the progeny RNP would be unidirectional, that is, NP is assembled either tail loop- or insertion groove-first. To test this, we performed competition assays between wild-type and mutant NPs during RNP reconstitution. Initially, the effect of NP concentration on viral replication and transcription was determined by titration ( Fig. 6a ). Conditions of limited NP concentration that allow detection of increasing or decreasing replication and transcription (transfection of 2 μg of wild-type NP-expressing plasmid, with 0.5 μg of each plasmid expressing polymerase subunits and 1,565-nucleotide-long RNA template) were selected. Next, increasing amounts of plasmid expressing oligomerization mutant NP, either R416A, E339A or E339A/R416A, were transfected with a constant amount of plasmid expressing wild-type NP, and the accumulation of viral RNA was analysed. As can be seen from Fig. 6b , the coexpression of NP with a mutation in the tail loop (NP R416A) had limited or no inhibitory effect on replication in the presence of wild-type NP, even when expressed in excess of wild-type NP. On the other hand, NP with a mutation in the insertion groove was highly dominant negative, inhibiting RNP activity even at a ratio of one in four relative to wild-type NP ( Fig. 6c ). However, the inclusion of a tail loop mutation (R416A) abrogated this strong inhibitory effect of the mutation in the insertion groove (E339A), as seen in Fig. 6d with double-mutant NP (E339A/R416A), resulting in only a limited inhibitory effect as observed with the R416A mutant alone. These data strongly suggest that NP joins the growing RNP unidirectionally in a tail loop-first orientation ( Fig. 6e ). NP R416A and NP E339A/R416A cannot be added to the growing RNP due to the mutation in the tail loop and are therefore non-competitive, although partial inhibition of RNP activity suggests limited competitive assembly of mutant NP into the RNP, possibly through non-oligomerization-mediated interaction with the RNP, for example, with the polymerase or RNA. On the other hand, the wild-type tail loop of NP E339A allows inclusion into the nascent RNP as efficiently as wild-type NP, but the mutation in its insertion groove prevents the assembly of further NP, resulting in loss of RNP activity. 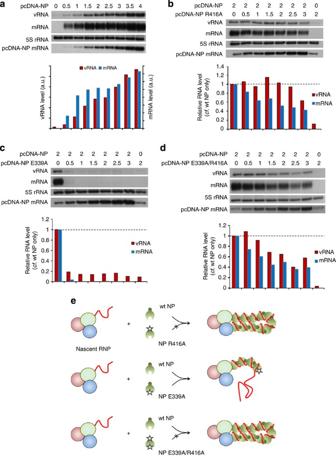Figure 6: Directionality of NP assembly onto RNP complexes. (a–d) The accumulation of vRNA and mRNA followingin vivoreconstitution of vRNPs from trimeric polymerase and full-length segment 5 vRNA in the presence of varying concentrations of wild-type (wt) NP (a) or wt and oligomerization mutant (R416A (b), E339A (c) or E339A/R416A (d)) NP was analysed by primer extension. A quantity of 0.5 μg of each of the polymerase subunit-expressing plasmids and the plasmid expressing the full-length segment 5 RNA template (containing mutations to prevent expression of NP) were transfected together with the amount of NP-expressing plasmid shown in μg (in a total of 6 μg (a) or 7 μg (b–d)). Analysis of the 5S rRNA levels served as an internal control. The level of mRNA derived from the NP-expressing plasmid is also shown. Quantification was performed by phosphorimage analysis. Graphs depicting the vRNA and mRNA levels accumulating in the presence of varying concentrations of wt and mutant NP relative to those accumulating in the presence of wt NP alone are shown. (e) Schematic depiction of competition assays demonstrating the directional assembly of NP onto nascent RNPs by homo-oligomerization. NP recruitment to the nascent RNP is mediated through NP homo-oligomerization, the tail loop of the incoming NP interacting with the insertion groove of the resident NP. Figure 6: Directionality of NP assembly onto RNP complexes. ( a – d ) The accumulation of vRNA and mRNA following in vivo reconstitution of vRNPs from trimeric polymerase and full-length segment 5 vRNA in the presence of varying concentrations of wild-type (wt) NP ( a ) or wt and oligomerization mutant (R416A ( b ), E339A ( c ) or E339A/R416A ( d )) NP was analysed by primer extension. A quantity of 0.5 μg of each of the polymerase subunit-expressing plasmids and the plasmid expressing the full-length segment 5 RNA template (containing mutations to prevent expression of NP) were transfected together with the amount of NP-expressing plasmid shown in μg (in a total of 6 μg ( a ) or 7 μg ( b – d )). Analysis of the 5S rRNA levels served as an internal control. The level of mRNA derived from the NP-expressing plasmid is also shown. Quantification was performed by phosphorimage analysis. Graphs depicting the vRNA and mRNA levels accumulating in the presence of varying concentrations of wt and mutant NP relative to those accumulating in the presence of wt NP alone are shown. ( e ) Schematic depiction of competition assays demonstrating the directional assembly of NP onto nascent RNPs by homo-oligomerization. NP recruitment to the nascent RNP is mediated through NP homo-oligomerization, the tail loop of the incoming NP interacting with the insertion groove of the resident NP. Full size image RNP complexes recruit NP independent of RNA binding To address whether homo-oligomerization between neighbouring NP molecules was mediated by RNA binding, or whether binding of NP to the RNA template follows homo-oligomerization-mediated recruitment, we constructed NP G1(4)/E339A by adding mutations in the RNA-binding groove to abolish RNA binding of the dominant-negative oligomerization mutant NP E339A. We hypothesized that a resultant loss of the dominant-negative phenotype in competition assays would suggest that RNA binding was a prerequisite for assembly of NP on the nascent RNP and homo-oligomerization. As a control, NP with mutations in the RNA-binding groove and the tail loop domain (NP G1(4)/R416A; Fig. 7a ) showed only weak inhibition in competition assays with wild-type NP. However, mutant NP G1(4)/E339A, despite reduced expression levels compared with wild-type NP ( Supplementary Fig. S3 ), retained a similar dominant-negative phenotype as NP E339A over wild-type NP ( Fig. 7b ). This implies that the loss of RNA binding had little impact on the ability of the NP E339A to assemble on the nascent RNP and to prevent the recruitment of further NP. Therefore, it appears that NP may be recruited to the nascent RNP through homo-oligomerization, independent of RNA binding, and that binding to the nascent RNA may occur subsequently ( Fig. 7c ). 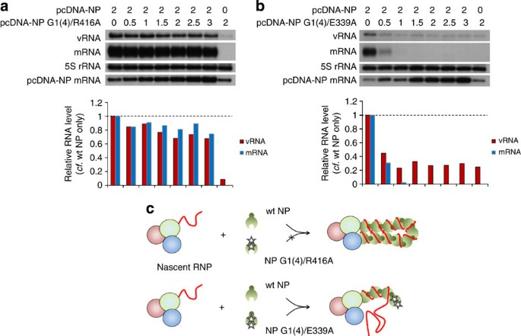Figure 7: The role of RNA-binding in recruitment of NP to RNP complexes. (a–b) The accumulation of vRNA and mRNA followingin vivoreconstitution of vRNPs from trimeric polymerase and full-length segment 5 vRNA in the presence of varying concentrations of wild type (wt) and dual RNA binding and oligomerization mutant (G1(4)/R416A (a) or G1(4)/E339A (b)) NP was analysed by primer extension. A quantity of 0.5 μg of each of the polymerase subunit-expressing plasmids and the plasmid expressing the full-length segment 5 RNA template (containing mutations to prevent expression of NP) were transfected together with the amount of NP-expressing plasmid shown in μg (in a total of 7 μg). Analysis of the 5S rRNA levels served as an internal control. The level of mRNA derived from the NP-expressing plasmid is also shown. Quantification was performed by phosphorimage analysis. Graphs depicting the vRNA and mRNA levels accumulating in the presence of varying concentrations of wt and mutant NP relative to those accumulating in the presence of wt NP alone are shown. (c) Schematic depiction of competition assays demonstrating the proposed RNA-binding-independent assembly of NP onto nascent full-length RNPs by homo-oligomerization. NP is recruited to the nascent RNP through docking of a wt tail loop to the wt insertion groove of the resident NP, independent of RNA binding. Binding to the nascent RNA may occur subsequently. Figure 7: The role of RNA-binding in recruitment of NP to RNP complexes. ( a – b ) The accumulation of vRNA and mRNA following in vivo reconstitution of vRNPs from trimeric polymerase and full-length segment 5 vRNA in the presence of varying concentrations of wild type (wt) and dual RNA binding and oligomerization mutant (G1(4)/R416A ( a ) or G1(4)/E339A ( b )) NP was analysed by primer extension. A quantity of 0.5 μg of each of the polymerase subunit-expressing plasmids and the plasmid expressing the full-length segment 5 RNA template (containing mutations to prevent expression of NP) were transfected together with the amount of NP-expressing plasmid shown in μg (in a total of 7 μg). Analysis of the 5S rRNA levels served as an internal control. The level of mRNA derived from the NP-expressing plasmid is also shown. Quantification was performed by phosphorimage analysis. Graphs depicting the vRNA and mRNA levels accumulating in the presence of varying concentrations of wt and mutant NP relative to those accumulating in the presence of wt NP alone are shown. ( c ) Schematic depiction of competition assays demonstrating the proposed RNA-binding-independent assembly of NP onto nascent full-length RNPs by homo-oligomerization. NP is recruited to the nascent RNP through docking of a wt tail loop to the wt insertion groove of the resident NP, independent of RNA binding. Binding to the nascent RNA may occur subsequently. Full size image Although it has previously been shown that the viral RNA polymerase is minimally sufficient for RNA synthesis from a short naked RNA template in vitro , NP has been found to be essential for replication and transcription of full-length genomic RNA in vitro and in vivo [20] , [22] , [23] , [24] , [40] , [41] . In the case of influenza A virus, short templates of 46 nucleotides have recently been found to be replicated in vivo in the absence of NP [21] . Here we have demonstrated that the influenza A virus polymerase is sufficient to carry out authentic in vivo replication and transcription of short vRNA-like templates efficiently in the absence of NP ( Fig. 1a ). Therefore, although NP has an important role in vRNP activity, it is not essential for determining the mode of initiation or termination of replication or transcription (capped primer initiated versus primer-independent initiation and termination with or without polyadenylation) by the viral polymerase or for the regulation of these activities. Instead, our findings demonstrate that template-associated NP represents an elongation factor that has a direct role in the stimulation of polymerase processivity, as has previously been proposed [20] . The latter model was based on in vitro data using virus-derived vRNPs stripped of NP. These authors suggested that the addition of NP facilitates escape of the viral polymerase from the promoter 12–19 nucleotides from the 3′-end. Similarly, NP of vesicular stomatitis virus, a non-segmented NSV, has recently been observed to be dispensable for in vitro synthesis of short RNA transcripts of approximately 21 nucleotides on naked RNA templates [42] . In contrast, we find that the influenza A virus polymerase is able to replicate vRNA templates of at least 76 nucleotides in the absence of NP in vivo , possibly implicating a cellular factor, such as the minichromosome maintenance complex [34] , in facilitating promoter escape of the polymerase in the absence of NP. We also find that the presence of NP promotes replication and transcription of very short templates, especially at low concentrations of polymerase ( Supplementary Fig. S2 ). Although we do not currently know the mechanism, it is possible that this reflects the multifunctional role of NP as a key adaptor molecule between virus and host cell processes [19] , [43] . For instance, NP may have a role through its interaction with the polymerase directly, either in the context of an RNP or free non-template-associated polymerase, in nuclear and cytoplasmic trafficking or indeed in polymerase activity. We also investigated the role of homo-oligomerization and RNA binding in RNP assembly and NP function. NP of H1N1 and H5N1 NP were both crystallized in trimeric form [13] , [14] , revealing the likely mode of interaction between neighbouring NP molecules in the RNP through the flexible tail loop structure [15] . Although the role of homo-oligomerization of NP is currently not known, it is generally thought to have a role in the assembly of RNPs. According to this model, NP is initially recruited to RNP through direct interaction with PB1 and PB2 of the polymerase bound to the nascent 5′-end of viral genomic or antigenomic RNA. Binding of subsequent NP to the RNA template may then be mediated by NP–NP homo-oligomerization [3] , [13] , [18] , [19] . However, homo-oligomerization has also been speculated to be RNA-mediated [15] , [44] , [45] , and oligomerization mutants of NP have previously been demonstrated to be impaired in RNA binding [46] . Indeed, surface plasmon resonance studies showed that although the RNA-binding affinities of oligomerization mutants NP R416A and NP E339A remained at submicromolar levels, their dissociation constants ( K D ) were about 60 times higher compared with wild-type NP (975 and 858 nM for NP R416A and NP E339A, respectively, compared with 15.8 nM for wild-type NP) [15] . This is likely to be due to oligomeric wild-type NP possessing more RNA-binding sites, contributing to a higher association rate and higher RNA affinity [15] . We discovered that the mutation in the insertion groove of NP (NP E339A), which prevents NP homo-oligomerization, has a dominant-negative phenotype in the assembly of a functional full-length wild-type RNP, whereas the mutation of the corresponding interactive residue in the tail loop (NP R416A) was non-competitive ( Fig. 6b ). It is unlikely that these results are related to differences in RNA-binding affinities between mutant and wild-type NPs, as the two oligomerization mutants have similar RNA-binding affinities [15] and similar phenotypes in supporting replication of intermediate-length templates ( Fig. 2b ) and in stabilizing full-length cRNA [29] , but have opposite effects in competition assays with wild-type NP. In addition, the dominant-negative phenotype of the insertion groove mutant NP E339A is abrogated by the introduction of the mutation (R416A) in the tail loop ( Fig. 6d ), whereas the addition of mutations in the RNA-binding groove of NP E339A had little effect on the dominant-negative phenotype ( Fig. 7b ). Therefore, we suggest that NP recruitment to the nascent RNP is mediated through NP homo-oligomerization, the tail loop of the incoming NP interacting with the insertion groove of the resident NP. In similar experiments, Shen et al. [47] found that mutant NP lacking the tail loop was uncompetitive in wild-type NP-supported transcription of a luciferase reporter gene in agreement with our data, whereas, surprisingly, both NP with the R416A tail loop mutation and E339A insertion groove mutation were dominant negative. Although the reason for this discrepancy is not clear, it may relate to these authors’ use of tagged NP. Nonetheless, these authors show the importance of the R416-E339 salt bridge for RNP assembly and activity during viral replication and the potential for antiviral drugs targeting this interaction. Our description of tail loop-first association of influenza A virus NP on nascent RNA is highly reminiscent of the directionality of NP of non-segmented NSVs revealed by the crystal structures of RNP complexes [48] , [49] and allows deduction of the orientation of the RNA strand in the vRNP structures published while this manuscript was under review [50] , [51] . We further determined that NP recruitment to the nascent RNP is not primarily mediated by RNA binding ( Fig. 7a ). Instead, we propose that NP is recruited by homo-oligomerization as described above, hypothetically followed by RNA binding, thereby stabilizing the nascent RNP and maintaining a continuously unfolded RNA template to facilitate replication. However, this raises the question of how homo-oligomerization mutants are recruited to nascent full-length RNA to form inactive but stable RNPs as shown previously [29] , or to form functional RNPs up to 221 nucleotides in length as shown here ( Fig. 2a–c ). As pointed out earlier, the efficiency of oligomerization mutant NP assembly into RNPs is dependent on the concentration of NP ( Supplementary Fig. S5 ). We propose that NP can be recruited to nascent RNP in an oligomerization-independent manner, possibly through interaction with the polymerase and/or the RNA template, when present in sufficient concentration, thereby stabilizing even full-length RNPs [29] ( Fig. 8 ). However, we suggest that non-oligomerizing NP recruited in this fashion only supports replication of intermediate-length templates up to approximately 250 nucleotides in length, either because of insufficient assembly of monomeric NP onto longer transcripts or because of a role for NP homo-oligomerization in modulating RNP template function beyond its role in RNP assembly. For instance, homo-oligomerization may have an additional role to enable transient displacement and repositioning of the NP on the template during the passage of the polymerase. 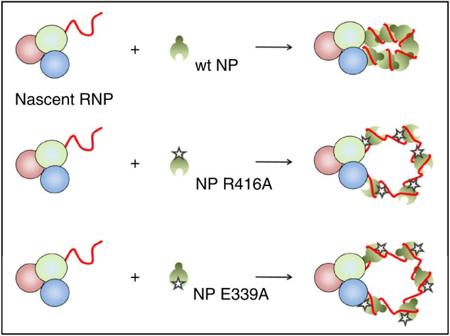Figure 8: Model for the recruitment of monomeric NP to RNP-like complexes. Schematic depiction of the proposed assembly of RNP-like complexes containing wild type (wt) or oligomerization mutant NP. Recruitment of wt NP to nascent RNP-like complexes is mediated through homo-oligomerization, whereas oligomerization mutant NP is recruited through polymerase- and/or RNA binding. The assembly of RNP-like complexes containing oligomerization mutant NP is more sensitive to the concentration of NP than the assembly of RNP-like complexes containing wt NP. Figure 8: Model for the recruitment of monomeric NP to RNP-like complexes. Schematic depiction of the proposed assembly of RNP-like complexes containing wild type (wt) or oligomerization mutant NP. Recruitment of wt NP to nascent RNP-like complexes is mediated through homo-oligomerization, whereas oligomerization mutant NP is recruited through polymerase- and/or RNA binding. The assembly of RNP-like complexes containing oligomerization mutant NP is more sensitive to the concentration of NP than the assembly of RNP-like complexes containing wt NP. Full size image In summary, we have shown here that NP of influenza A virus does not regulate the initiation or termination of transcription and replication. Instead, it supports the progress of the polymerase during the elongation phase. We have also shown that NP is unidirectionally recruited to nascent RNPs through homo-oligomerization and independently of RNA binding. The assays we have developed should allow more detailed investigation into the role of NP and the mechanisms of RNP replication and transcription. Furthermore, the approach described here to study the function and assembly mechanism of NP in influenza A virus RNPs should be readily adaptable to other NSVs. It will be interesting to determine the extent to which the polymerases of other NSVs are able to replicate and transcribe short vRNA-like templates in the absence of NP in vivo and the extent to which assembly mechanisms of NP onto nascent RNPs are conserved. Cells and plasmids Human embryonic kidney 293T cells were cultured in DMEM supplemented with 10% FCS. Plasmids expressing the PB2, PB1, PB1a (D445A/D446A), PA, PA-His 6 and NP proteins of influenza A virus A/WSN/33 (pcDNA-PB2, pcDNA-PB1, pcDNA-PB1a, pcDNA-PA, pcDNA-PA-His6 and pcDNA-NP) have been described previously [28] , [52] , as have plasmids expressing NP G1(4) (R74A/R75A/R174A/R175A), NP R416A and NP E339A (pcDNA-NP G1(4), pcDNA-NP R416A and pcDNA-NP E339A) [29] , and the vRNA expressing plasmids pPOLI-NP-RT and pPOLI-NS-RT [35] . Internal deletion mutants of pPOLI-NP-RT and pPOLI-NS-RT ( Supplementary Fig. S1 ) were made by round-the-plasmid PCR amplification, using two primers outwardly directed on the segment 5 or 8 gene sequence. PCR products were digested with SpeI and circularized by ligation. The NP open reading frame in the plasmid expressing full-length (1,565 nucleotides) segment 5 vRNA template was modified by site-directed mutagenesis, thereby eliminating the NP start codon (M1S) and introducing a stop codon (M238stop), to prevent expression of NP from transcribed mRNA. Plasmids expressing NP with mutations in both the oligomerization and/or RNA-binding domains (pcDNA-NP E339A/R416A, pcDNA-NP G1(4)/R416A and pcDNA-NP G1(4)/E339A) were constructed as chimeras from the individual mutants by restriction enzyme-mediated subcloning. Expression levels of mutant NP in transfected 293T cells were mostly comparable with wild-type NP, with the exception of NP G1(4)/E339A, which exhibited reduced accumulation ( Supplementary Fig. S3 ). The subcellular localization pattern of mutant NP compared with wild-type NP in transfected 293T cells was determined by immunofluorescence microscopy ( Supplementary Fig. S4 ). In vivo vRNP reconstitution One-millilitre suspensions of 293T cells (~10 6 cells) in DMEM supplemented with 10% FCS were transfected in 35 mm dishes using 1 μl of Lipofectamine 2000 (Invitrogen) per microgram of plasmid mixed with 150 μl OPTIMEM (Invitrogen). One microgram of each of the pcDNA plasmids expressing the polymerase subunits and NP, together with 1 μg of the pPOLI plasmid expressing the template RNA were transfected (in a total of 5 μg), except where indicated otherwise. Transfected DNA quantities in each experiment were kept constant by supplementing with pcDNA3A empty vector where necessary. Cells were collected 28 to 40 h post transfection. RNA isolation and primer extension analysis Total RNA was extracted from 10 6 transfected 293T cells with 1 ml Trizol (Invitrogen). One out of thirty μl of each RNA sample was mixed with an excess of 32 P-labelled DNA primers designed to detect negative and positive sense RNA of the different templates ( Supplementary Table S1 ) in 5 μl and denatured by heating at 95 °C for 5 min. The mixture was cooled on ice and transferred to 50 °C for 1 min before the addition of 5 μl 2 × transcription mix (2 × First Strand Buffer (Invitrogen), 20 mM dithiothreitol, 1 mM dNTP mix and 50 U SuperScript III RNase H−reverse transcriptase (Invitrogen)) also heated to 50 °C. The reaction was stopped after 1 h by the addition of 8 μl 90% formamide, and heating at 95 °C for 5 min. Transcription products were separated on 12% polyacrylamide gels containing 7 M urea in tris-borate-EDTA buffer and detected by autoradiography with intensifying screens. The presence of the 5′-terminal capped extension (which is of variable length) on mRNA allows clear separation of the mRNA reverse transcripts from those of cRNA. The level of vRNA template derived from RNA polymerase I-driven transcription of the input plasmid was determined by the omission of a single subunit of the viral polymerase and set to zero. The accumulation of vRNA was used as a measure of replication efficiency as the level of cRNA detected was considered to be too weak above background to quantitate. Quantitation was done using a Fuji phosphorimager and analysed using AIDA densitometry software. Oligo(dT) chromatography Total RNA from 3 × 10 6 transfected 293T cells collected at 48 h post transfection was extracted with Trizol (Invitrogen) and denatured at 95 °C for 5 min. RNA was mixed with 5 mg oligo(dT) cellulose (Sigma) in 200 μl binding buffer (0.5 M NaCl, 10 mM Tris-HCl, pH 7.5) and incubated with agitation at room temperature for 1 h. Oligo(dT) cellulose was pelleted in a microcentrifuge for 10 s and the supernatant (representing the unbound poly(A)–RNA fraction) was collected. The pellet was washed twice in binding buffer (1 ml) at room temperature, followed by incubation in 0.2 ml of low-salt buffer (0.25 M NaCl, 10 mM Tris-HCl, pH 7.5) at 37 °C for 15 min and repelleting. After washing the pellet with an additional 0.2 ml of low-salt buffer, the bound poly(A)+ RNA was eluted with 200 μl pre-warmed RNase-free water by incubating at 50 °C for 15 min and repelleting. The poly(A)+ and poly(A)− RNA fractions were recovered by Trizol extraction. Nickel-agarose affinity isolation of his-tagged RNP complexes Cell culture dishes (10 cm) of 293T cells were transfected as before using 9 μg of each plasmid (pcDNA-PB1, pcDNA-PB2, pcDNA-PA or pcDNA-PA-His6, pcDNA-NP or pcDNA-NP R416A and pPOLI-NP221) and 67.5 μl Lipofectamine 2000 (Invitrogen). Cells were collected 30 h post transfection, lysed in 1.5 ml of Tris-lysis buffer (50 mM Tris-HCl (pH 8.0), 200 mM NaCl, 20 mM imidazole, 33% glycerol, 0.5% Igepal CA-630, 1 mM dithiothreitol and 1 × complete mini EDTA-free protease inhibitor cocktail tablet) at 4 °C for 1 h, and centrifuged at 13,000 r.p.m. for 5 min. The cell lysate was then diluted 1 in 5 in Ni-agarose binding buffer (20 mM Tris-HCl (pH 8.0), 200 mM NaCl, 20 mM imidazole, 1 mM MgCl2 and 1 × complete mini EDTA-free protease inhibitor cocktail tablet) and incubated with 50 μl Ni-NTA agarose (Qiagen) for 4 h at 4 °C. The Ni-NTA agarose was washed five times in wash buffer (20 mM Tris-HCl (pH 8.0), 200 mM NaCl, 20 mM imidazole, 1 mM MgCl 2 , 10% glycerol, 0.1% Igepal CA-630). The Ni-NTA agarose was incubated at 4 °C for 2 h in 800 μl elution buffer (Ni-agarose wash buffer with 250 mM imidazole) and pelleted at 13,000 r.p.m. for 5 min. The supernatant was analysed by western blotting. Western blotting Transfected 293T cells were washed in 1 ml PBS. Twenty-five percent was resuspended in lysis buffer (250 mM Tris-HCl pH6.8, 2% SDS, 20% glycerol, 1.44 M β-mercaptoethanol) and the remaining 75% was used for RNA extraction. Cell lysates were analysed by SDS–PAGE followed by western blotting. Rabbit polyclonal antibody recognizing NP (1:10,000) was a kind gift from O. Haller. Rabbit polyclonal anti-PB1 (1:500), anti-RanBP5 (1:500) (Santa Cruz Biotechnology, Santa Cruz) or anti-beta actin (1:500) (Abcam, Cambridge) antibodies were used for loading controls. Immunofluorescence microscopy Vero cells grown on 13-mm coverslips in 24-well plates were transfected as ~70% confluent monolayers with 1 μg of expression plasmid and 1 μl of Lipofectamine 2000. The cells were incubated for 24 h, then washed with PBS and fixed with 4% paraformaldehyde in 250 mM HEPES (pH 7.5) for 15 min at room temperature. The cells were then permeabilized with 0.5% Triton X-100 in PBS for 15 min at room temperature, blocked overnight at 4 °C in blocking solution (PBS containing 1% BSA and 0.2% gelatine pH 8.0) and incubated with a rabbit polyclonal antibody recognizing NP (1:20,000; a gift from O. Haller) in blocking solution for 1 h at room temperature. Cy3-conjugated anti-rabbit (1:500) was used as the secondary antibody. Coverslips were mounted in Mowiol containing 0.001% 4′,6-diamidino-2-phenylindole (Sigma). Cells were viewed by using a Zeiss microscope with a Zeiss × 63/1.25 oil immersion objective, and the images were processed using ImageJ. How to cite this article : Turrell, L. et al. The role and assembly mechanism of nucleoprotein in influenza A virus ribonucleoprotein complexes. Nat. Commun. 4:1591 doi: 10.1038/ncomms2589 (2013).